Brønsted acid sites based on penta-coordinated aluminum species Zeolites and amorphous silica-alumina (ASA), which both provide Brønsted acid sites (BASs), are the most extensively used solid acid catalysts in the chemical industry. It is widely believed that BASs consist only of tetra-coordinated aluminum sites (Al IV ) with bridging OH groups in zeolites or nearby silanols on ASA surfaces. Here we report the direct observation in ASA of a new type of BAS based on penta-coordinated aluminum species (Al V ) by 27 Al-{ 1 H} dipolar-mediated correlation two-dimensional NMR experiments at high magnetic field under magic-angle spinning. Both BAS-Al IV and -Al V show a similar acidity to protonate probe molecular ammonia. The quantitative evaluation of 1 H and 27 Al sites demonstrates that BAS-Al V co-exists with BAS-Al IV rather than replaces it, which opens new avenues for strongly enhancing the acidity of these popular solid acids. The need for efficient and environmentally benign chemical processes has forced the replacement of harmful and corrosive liquid acids by solid acids in various fields of catalysis, including fine chemistry [1] , [2] , [3] , renewable energy production [4] , [5] , [6] , oil refining and petrochemical industries [7] , [8] . Silicon- and aluminum-based mixed oxides provide moderate and strong Brønsted acidity and are among the most popular solid acids used in current chemical processes [7] , [9] . Briefly, the solid acid catalysts can protonate hydrocarbon molecules to form carbocations and drive important reactions, such as cracking, hydrocracking, isomerization, alkylation and aromatization [10] , [11] , [12] , [13] , [14] , through surface complexes or transition states [15] . Crystalline zeolites and amorphous silica-alumina (ASA) are two main types of solid acids that contain Brønsted acid sites (BASs). It has been widely believed that only tetra-coordinated aluminum (Al IV ) atoms are able to contribute to the formation of BASs in nature [16] . In crystalline zeolites, the BASs are formed by protons, which compensate the negatively charged oxygens induced by the substitution of Si atoms by Al IV in the framework. The structure of these sites is well known as the bridging Si(OH)Al IV model ( Fig. 1a ) [15] , [16] , [17] . Replacing Si atoms by more Al IV species can enhance the density of BASs, but it reduces the mean electronegativity of the framework, which thus leads to a decrease of the overall acid strength of BASs [18] , [19] . Similarly, Al IV species incorporated into the amorphous silica network are able to generate BASs on ASA [9] , [20] , [21] . The proximity between Al IV and silanol sites in ASA has recently been observed by nuclear magnetic resonance (NMR) correlation experiments between 29 Si and 27 Al nuclei, the sensitivity of which was enhanced by dynamic nuclear polarization [22] . However, the strength of these BASs is generally lower than that on crystalline zeolites [7] and thus the presence of bridging OH groups ( Fig. 1a ) in ASA is still strongly under debate [22] , [23] . 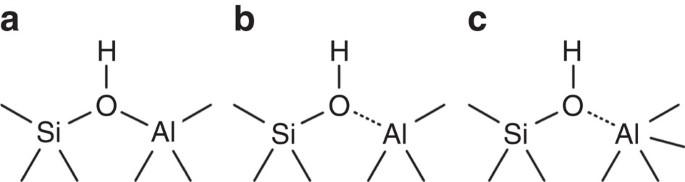Figure 1: Proposed models for BASs in silica-alumina catalysts. (a) BAS consisting of a bridging silanol site bonded to AlIVsite (Si(OH)Al) in zeolites15. (b) BAS consisting of the flexible coordination between silanol oxygen and neighbouring AlIV(ref.24). (c) BAS consisting of PBS interacting with AlIVsite27. In that later case, the dotted line does not denote a covalent bond but only the close proximity between O and Al atoms. Figure 1: Proposed models for BASs in silica-alumina catalysts. ( a ) BAS consisting of a bridging silanol site bonded to Al IV site (Si(OH)Al) in zeolites [15] . ( b ) BAS consisting of the flexible coordination between silanol oxygen and neighbouring Al IV (ref. 24 ). ( c ) BAS consisting of PBS interacting with Al IV site [27] . In that later case, the dotted line does not denote a covalent bond but only the close proximity between O and Al atoms. Full size image A flexible coordination between the Al IV atom and the neighbouring silanol oxygen atom ( Fig. 1b ) [9] , [21] , [24] , [25] or a pseudobridging silanol (PBS) with a nearby Al atom ( Fig. 1c ) [26] , [27] have been proposed [22] , to account for the longer Al-O distances (2.94–4.43 Å) in ASA [26] , with respect to those in the crystalline zeolite framework (1.88–2.0 Å) [28] . So far, most efforts focus on tuning the concentration of Al IV as the main route to increase the Brønsted acidity on zeolites or silica-alumina [29] , [30] , [31] , [32] , [33] . However, Al IV species tend to condense, to form an alumina phase at high Al/Si ratios [34] , [35] , [36] , leading to the decrease of Brønsted acidity. For ASA containing solely BASs based on Al IV species (BAS-Al IV ), the maximum Brønsted acidity has been obtained at 30 wt% Al loading [37] , [38] . In spite of the different BAS models, only Al IV species have been experimentally confirmed to contribute to the formation of BASs in these catalysts. Al V and Al VI species have been shown to act as Lewis acid sites on ASA and zeolites, but, to the best of our knowledge, no experimental evidence of BASs involving these sites has been reported so far [39] , [40] , [41] , [42] . Herein, we provide the direct experimental evidence for a new type of BAS-Al V in ASA by dipolar-mediated heteronuclear multiple quantum correlation ( D -HMQC) two-dimensional (2D) NMR experiments, which allow the detection of protons via 27 Al nuclei, hereafter noted 27 Al-{ 1 H}, hence probing the spatial proximities between different Al species and surface protons [43] , [44] , [45] . These experiments show that ASA can contain a large amount of Al V species located near SiOH groups. The acidity of these surface BAS-Al V sites has been demonstrated in this research by the adsorption of basic ammonia molecules, which react with BAS-Al V to form surface ammonium ions. Probing the connectivity between Al V species and SiOH groups The ASAs used in this work (see Supplementary Methods ) have been prepared according to a previously described procedure [9] , which generates ASA nanoparticles with a large amount of Al V species. The ASA powders are designated as SA/ X , where X is 10 or 50, indicating the molar fraction of Al in the precursor with respect to the total amount of Al and Si atoms. The obtained ASAs have tunable BAS acidity strengths ranging from moderate (SA/10 has an acidity close to zeolite H-X) to large (SA/30–70 have stronger BASs than zeolites H-Y and ZSM-5), depending on the aluminum content, as confirmed by both 13 C magic angle spinning (MAS) NMR investigation with probe molecule acetone and ammonia-temperature program desorption (TPD) [9] . The ASAs exhibited excellent catalytic performances for the conversion of phenylglyoxal with various alcohols, better than that of dealuminated zeolite Y, which hitherto was considered to be the most active solid acid in phenylglyoxal conversion [2] . The formation of BAS requires the aluminum atoms to be close to SiOH groups. Such proximity induces a dipolar coupling between 27 Al and 1 H nuclei, which can efficiently be probed by D -HMQC NMR 2D experiments based on coherence transfers via the 1 H- 27 Al dipolar couplings [46] , [47] . As shown in Fig. 2 , the correlation at δ 27A =50 p.p.m. and δ 1H =1.9 p.p.m. in the 27 Al-{ 1 H} D -HMQC 2D spectrum of dehydrated SA/50 indicates a close proximity between Al IV species and the proton of SiOH groups. This correlation is ascribed to the Si-OH···Al IV coordination: the typical BAS-Al IV often described for ASA ( Fig. 1c ) [16] . A very weak correlation at δ 27Al =10 p.p.m. and δ 1H =1.1 p.p.m. is assigned to the non-acidic terminal Al VI OH groups often observed on the surface of silica-alumina or zeolites, whereas the low-field broad hump at ca . 6 p.p.m. in the 1 H dimension could be caused by the small fraction of hydrogen-bonded AlOH groups [16] . Nevertheless, the most intense correlation is observed between Al V species ( δ 27A =30 p.p.m.) and SiOH protons ( δ 1H =1.9 p.p.m. ), which indicates the close proximity between SiOH groups and Al V species, and the presence of Si-OH···Al V coordination ( Fig. 2 ) in dehydrated SA/50. 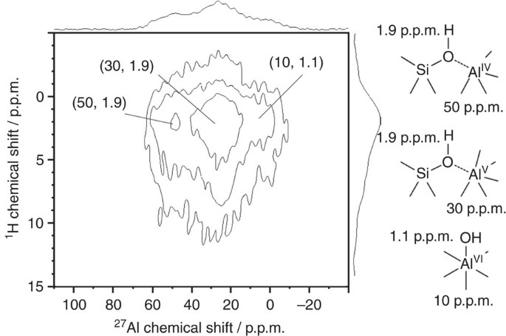Figure 2:27Al-{1H}D-HMQC 2D spectrum of SA/50. The sample was dehydrated at 723 K for 12 h under vacuum and recorded at 18.8 T with a MAS frequency ofνR=20 kHz andτrec=1.0 ms. The spectrum reveals that the proximity between SiOH groups and AlVspecies is dominant. Figure 2: 27 Al-{ 1 H} D -HMQC 2D spectrum of SA/50 . The sample was dehydrated at 723 K for 12 h under vacuum and recorded at 18.8 T with a MAS frequency of ν R =20 kHz and τ rec =1.0 ms. The spectrum reveals that the proximity between SiOH groups and Al V species is dominant. Full size image Al V -based BASs In zeolites, the substitution of a framework Si atom by an Al IV one to form one SiOHAl acid site ( Fig. 1a ) can shift the 1 H NMR signal of SiOH from ca . 1.8 to 3.6–5.2 p.p.m. (ref. 16 ). For these catalysts, BAS could be directly evidenced by the cross-peak in 27 Al-{ 1 H} D -HMQC 2D spectrum between Al IV species ( δ 27Al =60 p.p.m.) and the bridging OH groups ( δ 1H =4.3 p.p.m.) [43] . However, previous works have shown that the Al atoms with neighbouring SiOH groups ( Fig. 1b,c ) do not produce such a shift of the 1 H MAS signal of these groups [5] , [6] , [9] , [16] , [20] , [21] . Supplementary Fig. 1a,b show that the 1 H signal of SA/10 and SA/50 is centred around 1.9 p.p.m., thus indicating a majority of flexible or PBS coordination rather than zeolitic bridging coordination between SiOH groups and either Al IV or Al V species. Experiments using probe molecules have confirmed the role of flexible or PBS Si-OH···Al IV coordination as BAS in ASA [5] , [6] , [9] , [16] , [20] , [21] . Similar methods using ammonia probe molecules were applied here to demonstrate the acidity of the Si-OH···Al V coordination observed in dehydrated SA/10 and SA/50 (ref. 16 ). For these samples loaded with ammonia, the 1 H signal of ammonium ions was observed at δ 1H =6.7 p.p.m., as shown in Supplementary Fig. 1c,d , and commented in Supplementary Note 1 . The formation of these ions shows that ammonia reacts with BAS of SA/10 and SA/50. 27 Al-{ 1 H} D -HMQC experiments were also carried out to determine the nature of BAS, which protonate the ammonia molecules. Such a strategy based on 1 H- 27 Al correlations has been applied for [Al]MCM-41 loaded with ammonia. For such catalysts, ammonium ions ( δ 1H =6.7 p.p.m.) were only coupled to Al IV species ( δ 27A =56 p.p.m.) [44] . Hence, there was only evidence for BAS-Al IV on the surface of [Al]MCM-41, which protonated ammonia to ammonium ions. As seen in Fig. 3 , a correlation between NH 4 + ions ( δ 1H =6.7 p.p.m.) and Al IV ( δ 27Al =50 p.p.m.) is also observed in 27 Al-{ 1 H} D -HMQC spectra of SA/10 and SA/50, showing that the BAS-Al IV sites are also present on the surface of ASAs ( Fig. 4a ). Interestingly, these spectra also exhibit cross-peaks between Al V species ( δ 27Al =30 p.p.m.) and NH 4 + ions ( δ 1H =6.7 p.p.m.) in both SA/10 and SA/50. As seen in Fig. 3e , the intensity of this Al V -NH 4 + cross-peak is comparable to that of the Al IV -NH 4 + one. Given the BAS density ranging from 0.16 to 0.36 H + nm −2 in the investigated ASA samples ( Supplementary Table 1 ), each ammonia molecule only interacts with one BAS. The distance between the aluminum atom and the neighbouring silanol oxygen in ASA ranges from ca . 2.94 to 4.43 Å [26] and the N–H bond length in ammonia is only 1.02 Å [48] . As the heteronuclear coherence transfer in 27 Al-{ 1 H} D -HMQC is only effective up to a few angstroms, the protons of Si-O − (NH 4 ) + ···Al environment only interact with the neighbouring Al. The observation of an Al V -NH 4 + cross-peak in Fig. 3 at (30, 6.7) p.p.m. directly confirmed that ammonia is protonated on a BAS containing Al V : the Si-OH···Al V group. 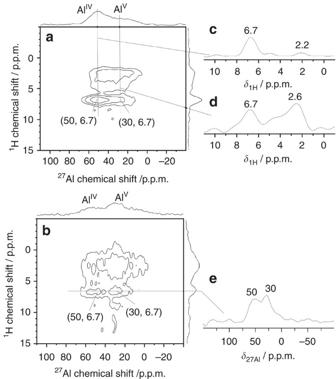Figure 3:27Al-{1H}D-HMQC 2D spectra of ammonia-loaded ASA samples. The dehydrated SA/10 (a) and SA/50 (b) samples were loaded with ammonia and evacuated at 373 K for 1 h, and the spectra were recorded at 18.8 T withνR=20 kHz andτrec=900 μs. The1H slices at the shifts of AlIVand AlVsites of SA/10 extracted from the 2D spectrum (a) are displayed in subfigures (c,d), respectively. The subfigure (e) shows the27Al slice at the shift of NH4+protons in SA/50 extracted from the spectrum (b). Figure 3: 27 Al-{ 1 H} D -HMQC 2D spectra of ammonia-loaded ASA samples. The dehydrated SA/10 ( a ) and SA/50 ( b ) samples were loaded with ammonia and evacuated at 373 K for 1 h, and the spectra were recorded at 18.8 T with ν R =20 kHz and τ rec =900 μs. The 1 H slices at the shifts of Al IV and Al V sites of SA/10 extracted from the 2D spectrum ( a ) are displayed in subfigures ( c , d ), respectively. The subfigure ( e ) shows the 27 Al slice at the shift of NH 4 + protons in SA/50 extracted from the spectrum ( b ). 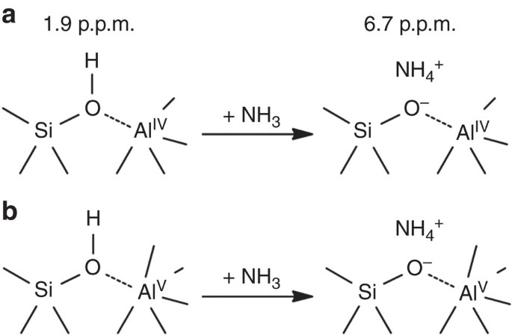Figure 4: Proposed proton transfer between BAS and ammonia molecules. (a) Ammonia protonated on conventional acidic BAS-AlIV. (b) BAS-AlVformed on ASA is able to transfer hydroxyl proton to ammonia, showing similar acidic properties as BAS-AlIV. Full size image Figure 4: Proposed proton transfer between BAS and ammonia molecules. ( a ) Ammonia protonated on conventional acidic BAS-Al IV . ( b ) BAS-Al V formed on ASA is able to transfer hydroxyl proton to ammonia, showing similar acidic properties as BAS-Al IV . Full size image The comparison of Supplementary Fig. 1c,d shows that more ammonia molecules are protonated on BAS-Al V in SA/50 than in SA/10. Combined with quantitative 1 H NMR investigations ( Supplementary Fig. 1 ) and the quadrupolar parameters ( Supplementary Table 2 and Supplementary Note 2 ) obtained from 27 Al one-dimensional MAS ( Supplementary Fig. 3 ) and 2D multiple quantum MAS ( Supplementary Fig. 2 ) NMR experiments, the analysis of 27 Al cross-peak intensities in 27 Al-{ 1 H} D -HMQC spectra ( Supplementary Fig. 4 and Supplementary Note 3 ) revealed that the population densities of both BAS-Al IV and -Al V on SA/50 (0.078 and 0.053 mmol g −1 ) were both higher than those of SA/10 (0.058 and 0.039 mmol g −1 ). This result suggests that BAS-Al IV and -Al V can co-exist on the surface rather than replacing each other and the population of both acid sites can be amplified by increasing Al content. Thus, this observation is promising for enhancing the population of BAS on ASA without limitation imposed by the Al contents. It should be noted that the F 2 projections of 27 Al-{ 1 H} D -HMQC 2D spectra are almost identical for dehydrated and ammonia-loaded SA/50 (see Supplementary Fig. 5 and Supplementary Note 4 ). Therefore, Si-OH···Al V and Si-OH···Al IV coordinations remained unchanged after the protonation of ammonia (as shown in Fig. 4 ). No Si-OH···Al IV have been transferred to Si-OH-Al V permanently after the adsorption of ammonia. In other words, the NMR results do not show the formation of permanent covalent bridges between silicate and Al IV or Al V sites in ASA samples after the deprotonation of BAS reacting with ammonia. Ammonia partially interacting with surface Al IV or Al V sites ( Fig. 3b and Supplementary Fig. 6 ) was also observed, which has been assigned to ammonia adsorbed on Lewis sites ( Supplementary Note 5 ). As shown in Fig. 1 , a surface bridging SiOHAl ( Fig. 1a ), a flexible coordination of SiOH and Al ( Fig. 1b ), or a pseudo-bridge between SiOH and Al atom ( Fig. 1c ) have been proposed for the formation of BAS-Al IV on ASAs. By analogy, similar structures might also contribute to the formation of BAS-Al V . The PBS model permits an explanation of the observation of the 1 H NMR signal of SiOH at 1.9 p.p.m. in both Fig. 2 and Supplementary Fig. 1 , whereas this 1 H signal of bridging OH groups ( Fig. 1a ) should occur at 3.6–5.2 p.p.m. If bridging OH groups are present in the investigated ASAs, their concentration must be below the limit of detection of the one-dimensional NMR MAS spectra of Supplementary Fig. 1 . Nevertheless, the current NMR data cannot rule out, in addition to PBS, the presence of bridging silanol groups in low concentration in ASA samples. These elusive strong BASs may also contribute to the catalytic activity in spite of their low concentration. The identification of all catalytic BASs in ASAs is beyond the scope of the present study, which is mainly to report the existence of BASs based on Al V environments. A final assessment of the local structure of BAS-Al V will require further experimental and theoretical work. In summary, a new type of BAS-Al V has been directly observed by 27 Al-{ 1 H} D -HMQC NMR spectroscopy. Hitherto, it was widely accepted that Al V sites only provide Lewis acidity [39] , [40] , [41] , [42] , and that solely Al IV ones contribute to the formation of BASs in aluminosilicate. However, we prove here by NMR experiments that similar to Al IV sites, Al V ones interact with neighbouring SiOH groups in ASA and behave as BASs in agreement with the PBS model. BAS-Al IV and -Al V seem to be structurally similar and show comparable acidity to protonate ammonia. Finally, a very important implication emerging from this work is that both Al IV and Al V species can co-exist on the surface of ASA. This feature facilitates that the total population density of BAS can be increased up to 70% by increasing the Al content, an amount much higher than the maximum Al loading of ca . 30% at which maximum acidity on ASA containing exclusively BAS-Al IV is achieved [37] , [38] . Hence, our findings not only report the existence of a new type of BAS in nature, but also open new avenues for creating high-performance solid acid catalysts containing Al V species, which will be promising for sustainable oil-refining and many industrial chemical processes. 27 Al-{ 1 H} D -HMQC 2D experiment All NMR experiments were recorded on a Bruker Avance III 18.8 T ( 1 H Larmor frequency of 800 MHz) spectrometer equipped with a 3.2 mm double-resonance MAS probe, in which rotors were spun at ν R =20 kHz. In the D -HMQC sequence, we have detected the 27 Al nuclei to benefit from their fast longitudinal relaxation times and the 1 H- 27 Al dipolar couplings were reintroduced by applying a SR recoupling on the 1 H channel [49] . The 1 H radiofrequency amplitudes for the 90° pulses and the SR recoupling were equal to ν 1 =62.5 and 40 kHz, respectively. The central transition selective pulse lengths on 27 Al were 8 and 16 μs for 90° and 180° pulses, respectively, that is, radiofrequency field amplitude ν 1 =10 kHz. The total dipolar recoupling time, τ rec , ranged from 700 to 1,000 μs depending on the sample. The 2D spectra resulted from the accumulation of 512 transients for each of 20 t 1 increments with Δ t 1 =50 μs and a recycle delay=1 s, that is, a total experiment time of about 3 h. Additional details about NMR experiments are given in the Supplementary Methods . Data availability The data that support the findings of this study are available upon request from the corresponding author J.H. and J.-P.A. How to cite this article: Wang, Z. et al . Brønsted acid sites based on penta-coordinated aluminum species. Nat. Commun. 7, 13820 doi: 10.1038/ncomms13820 (2016). Publisher's note: Springer Nature remains neutral with regard to jurisdictional claims in published maps and institutional affiliations.